The carotid body as a putative therapeutic target for the treatment of neurogenic hypertension In the spontaneously hypertensive (SH) rat, hyperoxic inactivation of the carotid body (CB) produces a rapid and pronounced fall in both arterial pressure and renal sympathetic nerve activity (RSA). Here we show that CB de-afferentation through carotid sinus nerve denervation (CSD) reduces the overactive sympathetic activity in SH rats, providing an effective antihypertensive treatment. We demonstrate that CSD lowers RSA chronically and that this is accompanied by a depressor response in SH but not normotensive rats. The drop in blood pressure is not dependent on renal nerve integrity but mechanistically accompanied by a resetting of the RSA–baroreflex function curve, sensitization of the cardiac baroreflex, changes in renal excretory function and reduced T-lymphocyte infiltration. We further show that combined with renal denervation, CSD remains effective, producing a summative response indicative of an independent mechanism. Our findings indicate that CB de-afferentation is an effective means for robust and sustained sympathoinhibition, which could translate to patients with neurogenic hypertension. The causes of human essential hypertension remain unknown. It is established that in many patients, sympathetic nerve activity increases proportionately as hypertension develops and this may be a causative factor [1] , [2] , [3] , [4] , [5] , but it is unclear what triggers heightened sympathetic traffic (reviewed in ref. 6 ). Despite good pharmacological control of arterial pressure in most patients with essential hypertension, a significant proportion remain drug resistant or intolerant to medication [7] , [8] , and this has been highlighted as a growing problem [9] , [10] . This presents a significant clinical challenge and provides the motivation to discover novel ways to control arterial pressure. Recently, the role of the carotid body (CB) chemoreceptors in the pathophysiology of cardiovascular disease is gaining considerable interest [11] , [12] , [13] , [14] , [15] . The sympathoexcitation in both sleep apnoea and heart failure may originate from enhanced activity of the CB chemoreceptors [16] , [17] , [18] , [19] , [20] . In both human patients and animal models of hypertension, the CB chemoreflex-evoked sympathoexcitatory responses are enhanced [15] , [21] , [22] , [23] . However, the hypothesis that CB chemoreceptor drive has an important role in the pathogenesis and/or maintenance of high arterial pressure was undetermined until most recently. We found that in spontaneously hypertensive (SH) rats, carotid sinus nerve denervation (CSD) lowered arterial pressure by ~17 mm Hg, and that this was well maintained and tolerated [11] . These data are comparable to those in human hypertensive patients where inactivation of the CB with 100% oxygen reduced both arterial pressure and sympathetic activity [24] , supporting a causal role for peripheral chemoreceptors in the aetiology of neurogenic hypertension. On the basis of these data, and that CB resection has been performed and well tolerated for the treatment of dyspnoea in ~5,600 patients with asthma and chronic obstructive pulmonary disease (reviewed in ref. 14 ), we recently proposed that CB ablation may be an effective interventional strategy to control blood pressure in drug-resistant hypertensive patients [11] , [14] . To assess the mechanisms underlying the hypotensive effect of CSD, we have made direct long-term simultaneous recordings of blood pressure and renal sympathetic nerve activity (RSA) before and after CSD in conscious SH and Wistar rats. Given the current clinical interest and application of renal denervation (RD) in the treatment of drug-resistant hypertension [25] , [26] , [27] , [28] , [29] , we have characterized the interaction between CSD and RD in combination to establish the type of interaction: summative, occlusive or facilitatory. Given that T lymphocytes have been shown to contribute to both angiotensin II and neurally mediated chronic hypertension [30] , [31] , we have assessed immune function following CSD. Unlike Wistar rats, we find that the CB of the SH rat has resting tone driving hypertension, which is not dependent on renal nerves, depresses both the cardiac and sympathetic vasomotor baroreflex and attenuates the adaptive immune response. We hypothesize that these findings may translate to patients with neurogenic hypertension. Transient inactivation of CB activity with hyperoxia All numerical data are reported as mean±s.e.m., with statistical significance ( P <0.05) determined using two-way analysis of variance (repeated measures for within-subject comparison), followed with the Holm–Sidek post hoc test. In SH rats, exposure to 100% oxygen to inactivate the CB produced falls in both systolic blood pressure (SBP; −12±4 mm Hg, n =5, P =0.047) and RSA (−2.9±0.4 μV, n =5, P =0.019) but no consistent change in the heart rate (HR; Fig. 1 ). In stark contrast, pure oxygen was without significant effect on these variables when delivered to Wistar rats or SH rats after CSD ( Supplementary Fig. S1 ). These data provide evidence that in SH rats, tonic afferent activity emanating from the CB provides a potent drive for neurogenically mediated hypertension. 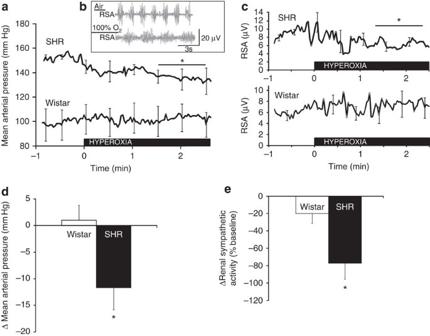Figure 1: The carotid bodies in hypertensive rats are tonically active. Comparing the effect of 100% oxygen to depress tonic CB activity in Wistar (n=6) and SH (n=6) rats on SBP (a) and RSA (b,c). The CB in SH rats, but not Wistar rats, exhibits tonic activity that is functionally relevant and contributes to basal arterial pressure (d) and sympathetic activity (e). Data are shown as mean±s.e.m. *P<0.05, repeated-measures analysis of variance. Figure 1: The carotid bodies in hypertensive rats are tonically active. Comparing the effect of 100% oxygen to depress tonic CB activity in Wistar ( n =6) and SH ( n =6) rats on SBP ( a ) and RSA ( b , c ). The CB in SH rats, but not Wistar rats, exhibits tonic activity that is functionally relevant and contributes to basal arterial pressure ( d ) and sympathetic activity ( e ). Data are shown as mean±s.e.m. * P <0.05, repeated-measures analysis of variance. Full size image Peripheral chemoreflex sensitivity in Wistar and SH rats Although previous studies have found increased reflex peripheral chemosensitivity in anaesthetized and decerebrate SH versus Wistar rats [15] , there are no data in conscious animals. Compared with Wistar rats, SH rats showed a more profound peripheral chemoreceptor reflex-evoked bradycardia (−194±5 versus −126±54 b.p.m., n =6, P =0.046) and RSA excitatory responses (13.4±0.8 versus 9±0.6 μV, n =6, P =0.021), but not a pressor response (54±8 versus 48±21 mm Hg; P =0.811) following an intravenous (i.v.) sodium cyanide bolus. Time profile of RSA response to CSD in SH and Wistar rats Following the surgery-related increase in RSA, there was a prompt and profound reduction in RSA below preoperative baseline after CSD in SH rats (−1.94±0.3 μV, −56±12%; n =6, P =0.027; Fig. 2a–c ). The peak fall occurred 5 days post CSD and showed no signs of recovery throughout the 3-week experimental period. The fall in RSA was correlated temporally with a fall in the mean arterial pressure of −17±3 mm Hg from a baseline of 137±7 mm Hg ( n =6, P =0.009). Spectral analysis also revealed a reduction in low-frequency (LF) SBP from 3.5±0.2 to 2.5±0.2 mm Hg 2 ( P <0.012; Table 1 ) suggesting a global reduction in sympathetic traffic. In these animals, we also tested the efficacy of CSD: Fig. 2d shows that the sympathoexcitatory reflex response following i.v. sodium cyanide was blunted severely. Despite the substantial fall in basal RSA after CSD, a stressful stimulus (high-frequency (HF) noise) continued to evoke a significant ( P =0.013) sympathoexcitatory response in SH rats, the magnitude of which was not different from those evoked before CSD (before: 139±28%, after: 153±13%, n =6, P =0.529; Fig. 2e ). This test served to both validate the viability of our chronic recordings and show that despite lower resting levels of RSA, alerting/arousal responses remained intact ensuring that fundamental visceral reactions were preserved. In Wistar rats, although there was no significant change in mean arterial pressure after CSD (−6±5 mm Hg, n =6), there was a small fall in RSA (−0.9±0.1 μV, −18±7%, n =6, P =0.045; Fig. 2a–c ), which was much less than that seen in SH rats ( P <0.01; Fig. 2a–c ). 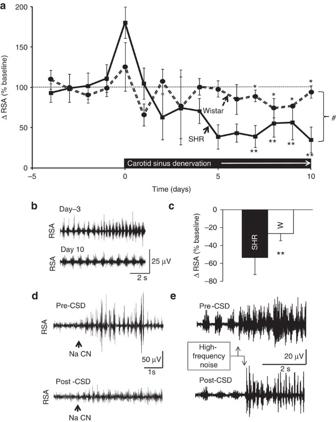Figure 2: Carotid sinus denervation causes substantial renal sympathoinhibition. Time profile of renal sympathetic nerve activity (RSA) response to bilateral carotid sinus nerve denervation (CSD) in SH (n=6) and Wistar (n=6) rats (a). Inset (b) shows the raw activity levels of RSA before and after CSD in one SH rat sitting quietly. The fall in RSA was ~55% relative to baseline in SH rats and significantly greater than that in Wistar rats (c). Efficacy of CSD is shown indwhere the sodium cyanide (i.v.)-evoked RSA excitatory response was greatly attenuated. (e) A CSD SH rat showing that it is able to generate a robust RSA response to a stressful stimulus. Data are shown as mean±s.e.m. *P<0.05, **P<0.01, between-groups analysis of variance (ANOVA);#P<0.05, repeated-measures ANOVA. Figure 2: Carotid sinus denervation causes substantial renal sympathoinhibition. Time profile of renal sympathetic nerve activity (RSA) response to bilateral carotid sinus nerve denervation (CSD) in SH ( n =6) and Wistar ( n =6) rats ( a ). Inset ( b ) shows the raw activity levels of RSA before and after CSD in one SH rat sitting quietly. The fall in RSA was ~55% relative to baseline in SH rats and significantly greater than that in Wistar rats ( c ). Efficacy of CSD is shown in d where the sodium cyanide (i.v. )-evoked RSA excitatory response was greatly attenuated. ( e ) A CSD SH rat showing that it is able to generate a robust RSA response to a stressful stimulus. Data are shown as mean±s.e.m. * P <0.05, ** P <0.01, between-groups analysis of variance (ANOVA); # P <0.05, repeated-measures ANOVA. Full size image Table 1 Cardiovascular and sympathetic effects of carotid sinus denervation. Full size table Baroreflex function improvement following CSD Cardiac baroreceptor reflex function curves were constructed recently after CSD [11] and showed an increase in sensitivity, which might contribute to the hypotensive effect of CSD; hence, we have analysed this in more detail. Consistent with this was the new finding that spontaneous cardiac baroreflex gain increased from −1.16±0.09 to −1.53±0.27 b.p.m. mm Hg −1 after CSD ( n =7, P <0.01). We also found an improvement in the sympathetic baroreflex sensitivity after CSD in SH rats ( Fig. 3 ), where the curve was shifted leftwards ( n =5, P =0.032) and the operating point moved to the left and downwards ( P =0.026; Fig. 3 ). An increase in the sensitivity of the curve was revealed by increases in both the upper and lower curvature parameters (see Supplementary Table S1 ), which translated into an increase in maximum gain (from −6.8±1.7 to −9.7±1.9% mm Hg −1 , P =0.028) towards that seen in Wistar rats (13.4±3.1% mm Hg −1 ). No significant changes in cardiac or sympathetic baroreflex function were found in Wistar rats post CSD ( Supplementary Fig. S2 ). 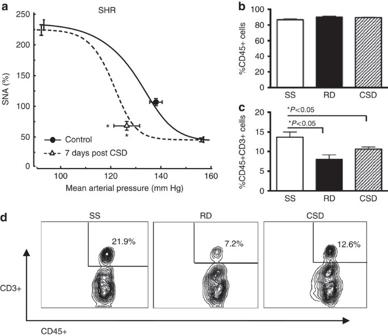Figure 3: Effects on the sympathetic baroreflex and vascular infiltration. (a) The renal sympathetic activity baroreflex function curve is rightwards shifted over lower pressure ranges after carotid sinus nerve denervation (CSD) in SH rats (n=6) but no changes were observed in Wistar rats (n=6,Supplementary Fig. S3). Percent total leukocytes (CD45+ cells) in the aorta of surgical sham (SS), RD and CSD animals (b). There was reduced vascular T-cell infiltration following RD and CSD in the SH rats as the percentage of T lymphocytes (CD45+CD3+ cells) in the aorta of RD and CSD animals was less relative to SS (n=6 and 7 per group;c). Representative flow cytometry contour plot showing T lymphocytes (CD45+CD3+) in aortic samples of each rat group (d). All data are shown as mean±s.e.m. *P<0.05, analysis of variance. Figure 3: Effects on the sympathetic baroreflex and vascular infiltration. ( a ) The renal sympathetic activity baroreflex function curve is rightwards shifted over lower pressure ranges after carotid sinus nerve denervation (CSD) in SH rats ( n =6) but no changes were observed in Wistar rats ( n =6, Supplementary Fig. S3 ). Percent total leukocytes (CD45+ cells) in the aorta of surgical sham (SS), RD and CSD animals ( b ). There was reduced vascular T-cell infiltration following RD and CSD in the SH rats as the percentage of T lymphocytes (CD45+CD3+ cells) in the aorta of RD and CSD animals was less relative to SS ( n =6 and 7 per group; c ). Representative flow cytometry contour plot showing T lymphocytes (CD45+CD3+) in aortic samples of each rat group ( d ). All data are shown as mean±s.e.m. * P <0.05, analysis of variance. Full size image Reduced T-cell infiltration into the aorta after CSD and RD Inflammation, in particular the adaptive immune response, has been shown to have a significant role in the pathogenesis of hypertension [30] , [31] , [32] . We therefore examined the effects of CSD and RD on the percentage of total aortic leukocytes (CD45+ average total cells 1.9 × 10 4 per aorta) and T lymphocytes (CD3+ average total cells 2.5 × 10 3 per aorta). The brainstem has also been identified as a site of increased inflammatory molecules during hypertension [33] , [34] ; therefore, we have examined the percentage of CD45+ CD3+ cells (average total cells 3.6 × 10 2 per brainstem) within this tissue. As shown in Fig. 3b , compared with the surgical shams there were no significant differences in the percentage of aortic CD45+ cells following CSD or RD procedures. However, when we examined the number of aortic infiltrates of CD3+ cells, there was a significant decrease in both CSD ( Fig. 3c,d ; P <0.01) and RD groups ( Fig. 3c–d ; P <0.01). Similarly, in single-cell suspensions of whole-brainstem homegenates, a significant reduction in percentage of CD3+ cells was determined following RD ( Supplementary Fig. S3 ; P <0.05) and a trend, which did not reach statistical significance, for a reduction in CD3+ cells in the CSD group. These data suggest that both CSD and RD procedures can reduce T-cell-mediated infiltration of tissue that has been associated with many forms of hypertension. Renal excretory function after CSD Given the alterations in arterial pressure and RSA, we looked to see whether renal function was altered. Despite our observed reduction in arterial pressure, SH rats showed an increase in 24-h urine volume at 12 days following CSD (from 4.25±0.28 to 5.57±0.32 ml/24 h/100 g body weight; P <0.05), which was sustained at days 21 and 28. This was accompanied by an increase in creatinine clearance (from 0.94±0.03 to 1.15±0.07 ml min −1 ; P <0.01), indicating an increase in glomerular filtration rate. The total protein in urine decreased significantly (from 10.5±1.0 to 8.7±0.8 mg ml −1 ; P <0.05), albuminuria was lower after CSD but not significant (from 0.57±0.05 to 0.45±0.05 mg ml −1 ; P =0.067), although water intake also increased significantly (from 10±1.2 to 12.8±1.6 ml/24 h/100g body weight; P <0.01). For comparison, Wistar rats had a lower total protein and albumin level in their urine compared with SH rats before denervation: 9.75±0.84 versus 10.49±0.77 mg ml −1 and 0.40±0.06 versus 0.57±0.05 mg ml −1 , respectively. The water intake and creatinine clearance was similar between Wistar and SH rats before denervation: 30.81±2.13 versus 30.49±2.13 ml/24 h and 0.83±0.07 versus 0.94±0.03 ml min −1 , respectively. Taken together, these data indicate that the progression of glomerular kidney damage/leakage in SH rats may have been retarded by CSD. Time to sympathoinhibition after CSD in SH rats In conscious SH rats, it was not possible to assess the precise time to onset of the depressor and sympathoinhibition following CSD because of the side effects of surgery and anaesthesia. To this end, we recorded internal cervical (iCSN) and lumbar sympathetic post-ganglionic nerves simultaneously before and after CSD in in situ -unanesthetized decerebrated SH rats. 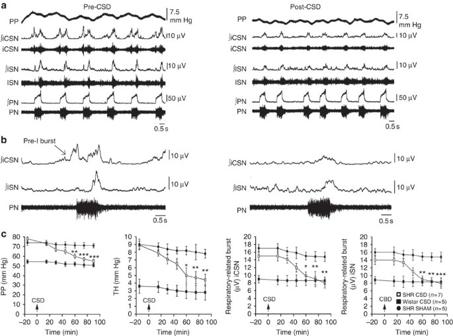Figure 4: Immediate effects of carotid sinus denervation. The time course of the fall in sympathetic nerve activity (raw and integrated) after carotid sinus nerve denervation (CSD) was compared for the internal cervical (iCSN) and lumbar (lSN) sympathetic post-ganglionic nervesin situ. By 40 min, there was a significant decrease in the sympathetic nerve activity in both outflows (a). Note the decrease in the amplitude of respiratory-modulated discharge (P<0.05;b). The peak response was achieved at 60 min post CSD as activity levels at 75 or 90 min were not different from the level recorded at 40 min post CSD but were different from their own baseline (c). Data are shown as mean±s.e.m. *P<0.05, **P<0.01, ***P<0.001, repeated-measures analysis of variance;n≥5. PN, phrenic nerve; PP, perfusion pressure (aortic); Pre-I, pre-inspiratory; TH, Traube–Hering arterial pressure waves. Figure 4 shows that by 40 min, there was already a significant decrease in sympathetic nerve activity in all outflows and that this was due, in part, to a decrease in the amplitude of respiratory-modulated discharge ( P <0.05; Fig. 4b ). The peak response was achieved at 60 min post CSD, as activity levels at 75 or 90 min were not different from the level recorded at 40 min post CSD but were different from their own baseline (both P <0.01; Fig. 4c ). Consistent with the reduction of respiratory-sympathetic modulation, we found a decrease in HF SBP in conscious SH rats after CSD (from 4.52±0.3 to 3.9±0.3 mm Hg 2 ; n =7, P <0.05). Figure 4: Immediate effects of carotid sinus denervation. The time course of the fall in sympathetic nerve activity (raw and integrated) after carotid sinus nerve denervation (CSD) was compared for the internal cervical (iCSN) and lumbar (lSN) sympathetic post-ganglionic nerves in situ . By 40 min, there was a significant decrease in the sympathetic nerve activity in both outflows ( a ). Note the decrease in the amplitude of respiratory-modulated discharge ( P <0.05; b ). The peak response was achieved at 60 min post CSD as activity levels at 75 or 90 min were not different from the level recorded at 40 min post CSD but were different from their own baseline ( c ). Data are shown as mean±s.e.m. * P <0.05, ** P <0.01, *** P <0.001, repeated-measures analysis of variance; n ≥5. PN, phrenic nerve; PP, perfusion pressure (aortic); Pre-I, pre-inspiratory; TH, Traube–Hering arterial pressure waves. Full size image Comparing uni- versus bilateral CSD in SH rats We wished to test any difference in the sympathoexcitatory drive from the left versus the right CB as well as their individual responses. 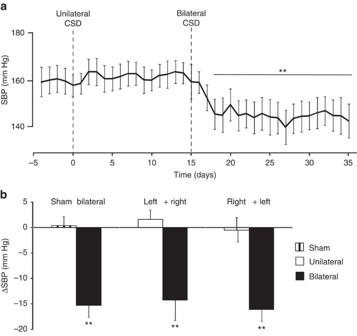Figure 5: Unilateral carotid sinus denervation does not lower blood pressure in the rat. Unilateral carotid sinus nerve denervation (CSD) was ineffective at lowering SBP in SH rats whether the left or right CB was removed (n=8;a). Irrespective of whether the left or right CB was removed first, there was no difference in the fall in SBP observed on removal of the contralateral CB (b). Note that time-staggered unilateral CB denervation does not affect the magnitude of the fall in SBP, which is the same as that seen when both left and right CB are denervated simultaneously (seeFigs 2,3). Data are shown as mean±s.e.m. **P<0.01, within-group analysis of variance. Figure 5 shows the time profile of the response in SBP following unilateral and subsequent bilateral CSD. Unilateral CSD, whether targeting the left ( n =4) or right side ( n =4) produced no change in SBP ( Supplementary Table S2 ). The fall in SBP achieved when bilateral CSD was staggered in time by 15 days (that is, denervating left then right CB, or denervating right then left CB) was no different from the response when both the CBs were denervated at the same time (−16±2 versus −17±3 mmHg, respectively, P =0.831). In our in situ preparation, which allowed high temporal resolution of changes in sympathetic activity (see above), unilateral CSD did not produce a measureable change in any of the recorded variables. Figure 5: Unilateral carotid sinus denervation does not lower blood pressure in the rat. Unilateral carotid sinus nerve denervation (CSD) was ineffective at lowering SBP in SH rats whether the left or right CB was removed ( n =8; a ). Irrespective of whether the left or right CB was removed first, there was no difference in the fall in SBP observed on removal of the contralateral CB ( b ). Note that time-staggered unilateral CB denervation does not affect the magnitude of the fall in SBP, which is the same as that seen when both left and right CB are denervated simultaneously (see Figs 2 , 3 ). Data are shown as mean±s.e.m. ** P <0.01, within-group analysis of variance. Full size image SBP response to combined CSD and RD Given the current interest in RD [25] , [26] , [27] , [28] , [29] , the relative potency and interaction (occlusive, summative and facilitatory) of RD versus CSD and was deemed scientifically and clinically important. All sham-operated SH rats showed a time-related increase in SBP (4±4 and 3±2 mm Hg for sham CSD–RD and sham RD–CSD, respectively; Figs 6 ). The efficacy of RD was confirmed by measuring renal noradrenaline content after RD (with or without concurrent CSD), which showed a significant reduction compared with sham controls (RD alone: 45±6; RD with CSD: 31±9; sham: 443±54 pg per 100 μg protein; n =18, P <0.01). The data reported herein are all expressed relative to the preoperative control level. 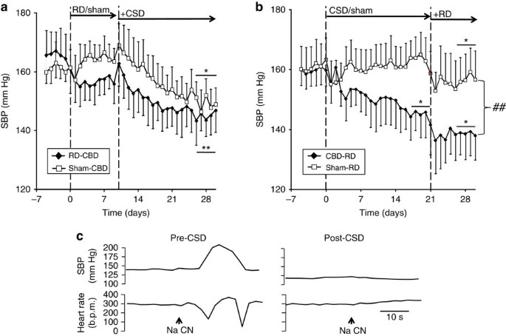Figure 6: Carotid sinus and RD interaction time course. Time profile of the SBP response to (a) renal nerve denervation (RD) followed by carotid sinus nerve denervation (CSD;n=6) and (b) CSD followed by RD resection in SH rats (n=7). Note the time-dependent increase in SBP in shams (n=6 and 7, respectively). The completeness of the CSD is shown by the absence of a reflex pressor and bradycardic response following i.v. injections of sodium cyanide (NaCN;c). Data are shown as mean±s.e.m., repeated-measures analysis of variance (ANOVA): *P<0.05, **P<0.01; between-group ANOVA,##P<0.01. Figure 6: Carotid sinus and RD interaction time course. Time profile of the SBP response to ( a ) renal nerve denervation (RD) followed by carotid sinus nerve denervation (CSD; n =6) and ( b ) CSD followed by RD resection in SH rats ( n =7). Note the time-dependent increase in SBP in shams ( n =6 and 7, respectively). The completeness of the CSD is shown by the absence of a reflex pressor and bradycardic response following i.v. injections of sodium cyanide (NaCN; c ). Data are shown as mean±s.e.m., repeated-measures analysis of variance (ANOVA): * P <0.05, ** P <0.01; between-group ANOVA, ## P <0.01. Full size image Figure 6 shows the time profile of the SBP response to RD followed by CSD ( Fig. 6a ) and CSD followed by RD ( Fig. 6b ). In SH rats, performing RD first produced a fall of SBP of −9±2 mm Hg from a baseline of 166±5 mm Hg ( n =6, P <0.013). A further fall of −12±3 mm Hg ensued after subsequent CSD ( P <0.001) and showed no recovery over the observational period. In SH rats undergoing the CSD–RD surgical sequence, basal SBP was 160±8 mm Hg, CSD alone evoked a prompt fall of −14±2 mm Hg ( n =7, P <0.001) with a further fall of −6±2 mm Hg ( P <0.001) after RD; no recovery was observed over the time course of the study. The total fall (−17±2 mm Hg) was not different from that measured with the reversed sequence of RD–CSD (−20±3 mm Hg; P =0.363). These data are summarized in Fig. 7 and show an additive interaction between RD and CSD that this is similar irrespective of the order in which the surgical procedures are carried out in SH rats. CSD, but not RD, produced significant bradycardia ( P =0.018) and a small reduction in respiratory frequency ( P <0.01) in SH rats ( Table 1 ). Table 1 documents spectral frequency analysis of both pulse interval and SBP after RD–CSD and CSD–RD. RD alone resulted in an increase in spontaneous baroreflex gain (−1.73±0.4 b.p.m. mm Hg −1 mmHg; P <0.01; Table 1 ) and decrease in CD3+ cells ( Fig. 3b–d ; P <0.01). Figure 6c demonstrates that the reflex bradycardia and pressor responses to sodium cyanide (i.v. ), used to activate peripheral chemoreceptors in conscious SH rats, were abolished after bilateral CSD. 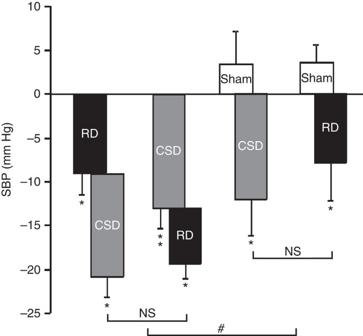Figure 7: Carotid sinus and RD interaction summary. Group data show the interaction between carotid sinus nerve denervation (CSD;n=6) and renal nerve denervation (RD;n=7) in SH rats. There was an additive effect of CSD and RD, irrespective of the order in which the intervention was made. The combined intervention produced a greater fall in SBP than each RD or CSD alone. Data are shown as mean±s.e.m., repeated-measures analysis of variance (ANOVA): *P<0.05, **P<0.01; between-group ANOVA,#P<0.05. Figure 7: Carotid sinus and RD interaction summary. Group data show the interaction between carotid sinus nerve denervation (CSD; n =6) and renal nerve denervation (RD; n =7) in SH rats. There was an additive effect of CSD and RD, irrespective of the order in which the intervention was made. The combined intervention produced a greater fall in SBP than each RD or CSD alone. Data are shown as mean±s.e.m., repeated-measures analysis of variance (ANOVA): * P <0.05, ** P <0.01; between-group ANOVA, # P <0.05. Full size image Our data demonstrate that the CB in the conscious SH rat is constitutively active and provides a tonic prohypertensive drive. Mechanistically, the antihypertensive effects of CSD in SH rats include a substantial reduction in sympathetic nerve discharge including that to the kidney, involving a reduction of respiratory modulation; a resetting of the sympathetic baroreflex over lower arterial pressures; an improvement in spontaneous cardiac baroreflex gain; possible changes in renal excretory function; and a reduction in vascular T-cell infiltration. Unilateral CSD, whether on the left or right side, was ineffective in reducing arterial pressure but subsequent resection of the contralateral side remained an effective antihypertensive therapy. In conscious SH rats, we show that CSD is more potent as an antihypertensive intervention than RD but that the renal nerves are not necessary for the hypotensive effect of CSD. Combining RD with CSD, or reversing the sequence (CSD then RD), gives an additive response that is similar in magnitude, irrespective of the order in which the surgical procedures are performed. RD in young SH rats prevents the full development of hypertension [35] , [36] . The fall in arterial pressure by ~9 mm Hg we report herein following RD in Wistar rats is consistent with previous studies in Sprague–Dawley rats [37] but not with Wistar–Kyoto rats, where arterial pressure was unaltered [35] , [38] . Previous reports in SH rats demonstrated larger falls in arterial pressure after RD (~19 mm Hg (refs 36,38)) [36] , [38] relative to our results (~9 mm Hg). The difference may reflect the use of tail cuff/indwelling catheters rather than radio-telemetry and between-group versus within-animal analyses. Despite these quantitative differences, renal nerves (afferent and/or efferent) have a tonic role in regulating arterial pressure in some strains of normotensive and SH rats, as reviewed recently [39] . In conscious SH rats, our finding that the CB chemoreflex sensitivity is elevated relative to the Wistar animal is consistent with prior data from animals and humans [15] , [21] , [22] , [23] . For the first time, we describe heightened CB tonicity in SH rats as revealed by a depressor and sympathoinhibitory response to hyperoxia in SH but not Wistar rats. This suggests that the CB has elevated activity in the SH rat providing excitatory drive to the generation of sympathetic vasomotor tone that in turn contributes to the hypertension, as recently described in hypertensive human patients [24] . It may also explain why CSD is effective in producing a long-term antihypertensive response. The tonic activity in SH rats may result from increased expression of ASIC3 and TASK1—two acid-sensing non-voltage-gated channels [15] . Others suggest that the balance between carbon monoxide and hydrogen sulphide within the CB and the activity of HIF-1α versus HIF-2α have a role [40] . Animal models of chronic heart failure have revealed that CB chemoreceptor activity is augmented by angiotensin II receptors [41] , impaired nitric oxide synthase activity [20] , reduced CB blood flow [42] , enhanced adenosine monophosphate-activated protein kinase [43] and inflammation [44] , [45] . Heightened sympathetic drive to the arterioles of the CB itself may also contribute to its hyperactivity because of hypoperfusion (via vasoconstriction and vascular remodelling [46] ) and inflammation. Because of the complications of anaesthesia and surgical recovery, we were unable to determine the precise time-dependent effects following CSD in conscious SH rats. Using our in situ rat preparation, a fall in perfusion pressure and sympathetic activity occurred at 40 min post CSD indicating a relatively rapid response. Presumably, 40 min permits a reconfiguration of the cardio-respiratory brainstem network in the in situ rat, as reflected by a reduction in both respiratory-sympathetic coupling and the magnitude of the Traube–Hering wave amplitude. Consistent with reduced respiratory-sympathetic coupling, we saw a decrease in HF SBP spectra in conscious SH rats after CSD. Given that respiratory-sympathetic coupling contributes significantly to vascular resistance and arterial pressure development the SH rat [47] , this could be a major mechanism for the CSD-evoked antihypertensive effect. It was evident that removal of a single CB, whether the left or right, in vivo or in situ , was ineffective in lowering arterial pressure in SH rats, although there was a brief reduction in respiratory frequency, perhaps indicative of a transient effect. Given that CB afferents terminate in the commissural nucleus tractus solitarious (NTS) with axons traversing the midline providing ample innervation of contralateral targets [48] , it perhaps is not surprising that unilateral CSD was not effective long-term. On subsequent removal of the second CB from a SH rat with chronic, unilateral CSD, arterial pressure fell precipitously; the level reached was not different from that recorded following a procedure where both CBs were removed at the same time. This suggests that any compensation occurring after loss of a single CB does not affect the efficacy of response following contralateral CB denervation. Whether these findings relate to humans with hypertension is unknown but provides two predictions. The first is that unilateral CSD may be effective transiently in lowering arterial pressure and compensated for with time. Second, subsequent CB resection following a unilateral procedure will cause a potent hypotensive effect. For safety reasons, a clinical study should start with unilateral CB ablation; thus, knowing that a hypotensive effect persists following staggered bilateral CSD (that is, not ameliorated by a prior unilateral intervention) is an important preclinical information. Previously, we have shown that CSD in young, prehypertensive SH rats prevented the full manifestation of hypertension and lowered arterial pressure in adult SH rats [11] . Using both power spectral analysis and hexamethonium to block ganglionic transmission, we provided indirect evidence that the hypotension was caused, in part, by a generalized reduction in sympathetic activity [11] . Here we demonstrate for the first time that the CSD-induced hypotension was accompanied with a substantial reduction in RSA that fell with a similar time course. Despite this robust reduction of ~55% in RSA, we showed that animals were not left sympathetically incompetent, and, importantly, could respond vigorously to a stressor stimulus. Given that lumbar and cervical sympathetic outflows also fell (as shown acutely), we suspect that there is widespread sympathoinhibition following CSD and that it is not confined to the kidneys. This is supported by a chronic reduction in LF spectra of SBP. This has important clinical implications regarding the applicability of CSD beyond hypertension to conditions such as heart failure, sleep apnoea and insulin resistance, where there is excessive and pathological sympathetic activity [14] . The mechanisms for blood pressure reduction following CSD are likely to be numerous and operate over different time scales giving a persistent effect. Our hyperoxia data clearly shows that removal of CB tone in SH rats can, at least acutely, provide sympathoinhibition. This may suggest a hypoxic drive within the CB of the SH rat, which might be the stimulus for the increased density of small vessels in the CB of SH versus normotensive rats [46] . However, we do not rule out non-hypoxic intra-CB drives to explain the tonicity within the SH rat CB. Other mechanisms by which CSD lowers blood pressure include an improvement in both cardiac and sympathetic vasomotor limbs of the baroreflex after CSD [11] . As our method of CSD removes innervation of the carotid sinus baroreceptors, the improvement in baroreceptor reflex function must be of aortic baroreceptor origin. On the basis of this observation, it is expected that selective removal of the CB, sparing carotid sinus baroreceptors, would be predicted to enhance their gain also and produce a greater antihypertensive effect. The known antagonistic interaction between chemo- and baro-afferents both centrally (at a neuronal level within nucleus tractus solitarii [49] ) and of their respective reflex responses [50] could explain this beneficial result as enhanced baroreflex function can contribute to the long-term lowering of blood pressure and sympathetic activity in dogs [51] and humans [52] . We do not rule out improved compliance of the aorta, central plasticity and/or improved cardiac vagal transmission to explain better baroreflex function after CSD in SH rats. The finding of reduced iCSN activity may improve the brainstem blood flow; given that the SH rat brainstem is hypoperfused, improving flow may contribute to reducing arterial pressure [53] . Our observation of increased urine production and glomerular filtration rate in the face of decreased systemic arterial pressure indicates that CSD may be associated with active improvements in renal excretory function. This may be mediated, at least in part, directly through the substantial inhibition of renal sympathetic activity and may contribute to the hypotensive effect of CSD through fluid excretion. The reduced percentage of vascular and brainstem infiltrates of T lymphocytes is unlikely to contribute to the prompt fall in the arterial pressure because of its rapid time course but may assist in the long-term maintenance of the hypotensive effect of CSD especially because T lymphocytes have been shown to contribute to both angiotensin II and neurally mediated chronic hypertension [54] , [55] . We speculate that the sympathoinhibitory effect of CSD contributes to reduced T-cell infiltration in the aorta and brainstem described herein, which could improve vascular compliance including the aortic baroreceptor sensitivity and improved baroreflex transmission centrally [33] , [34] . The location of the vascular immune cell infiltrates is unknown but we speculate based on previous studies [56] that these cells predominantly accumulate in the adventitia and perivascular adipose tissue of blood vessels. Given the sympathetic innervation of immune system organs such as the spleen, thymus and bone marrow [26] , we suggest that reductions in sympathetic activity may be the trigger for the anti-inflammatory response, thereby breaking this positive (and pathological) feedback loop [6] . One successful new antihypertensive interventional approach is RD, which appears to be a safe treatment in some humans with drug-resistant hypertension [25] , [26] , [27] , [28] , [29] . In one study, blood pressure was lowered by >10 mm Hg with a high success rate (84%), although all patients remained hypertensive and their antihypertensive medication was maintained [25] . In contrast, an 84% success rate was not confirmed by other groups who reported no overall change in the arterial pressure, although some individuals did respond [27] or around a 40–50% blood pressure response rate [26] , [28] , [29] . Given these findings, and the recent success of unilateral CB resection in a heart failure patient [57] , CB ablation to control arterial pressure in drug-resistant hypertensive patients could be considered. Thus, scenarios are imagined that include patients in which RD has not lowered arterial pressure to target levels; not circumvented prescribed and poorly tolerated medication; and failed and not been possible because of renal artery stenosis or bifurcation. Thus, it becomes critical to study any interaction on arterial pressure following combined RD and CSD as well as CSD alone procedures. The finding that unilateral CB resection in a heart failure patient was effective in correcting partially both cardiac autonomic balance and cardiac baroreflex gain [57] , yet ineffective in altering these variables in SH rats is curious. Clearly, heart failure and hypertension have distinct pathologies, which could explain this difference. Equally, there may be differences in CB signalling mechanisms between SH rats and humans that could contribute to response differences between unilateral versus bilateral CB resection. This remains an open question. In conclusion, there is an additive antihypotensive interaction between CSD and RD, which is unaffected by either the order or timing of the procedures. Bilateral CSD provides a potent and persistent antihypertensive response in SH rats accompanied by substantial sympathoinhibition in multiple outflows, improved baroreflex and renal function, and reduced T-lymphocyte infiltration in the aorta and brainstem. Whether CSD offers therapeutic benefit to drug-resistant/intolerant human patients with sympathetically mediated diseases is currently undergoing clinical trial. Renal and CB surgery Animal experiments were conducted in accordance with the UK Animals (Scientific Procedures) Act 1986 and associated guidelines and approved by the University of Bristol Ethics Committee. Adult male (12 weeks; n =38) SHR and Wistar rats (12 weeks; n =6) bred in the University of Bristol Animal Services Unit were used. For all surgeries, rats were anaesthetized with ketamine (60 mg kg −1 ; intramuscular) and medetomidine (250 μg kg −1 , intramuscular), and aseptic techniques were used. For CSD, the CB was approached via an anterior midline neck incision and the carotid sinus nerve branches were sectioned [11] . Sham-operated rats underwent the same surgical procedures to expose the CB but the carotid sinus nerves were left intact. Unilateral CSD rats (SH, n =8) were randomized to have either their left ( n =4) or right ( n =4) carotid sinus denervated first, followed by contralateral denervation 14 days later. On denervating the second CB, a transient apnoea occurred in all SH rats with some requiring resuscitation. This apnoea was not observed in Wistar rats. No post-surgical mortalities occurred, suggesting that there were no lethal apnoeic episodes post CSD and all rats gained weight normally. To assess the efficacy of CSD, arterial pressure was recorded (and from this, HR and respiratory frequency were derived) during an injection of sodium cyanide (NaCN, 100 μl 0.04% i.v.) 1–2 weeks post CSD. Bilateral RD was achieved via a retroperitoneal incision to allow retraction of each kidney and exposure of the renal artery. The nerves and adventitia were stripped from the renal artery and renal plexus, which were then painted with a dilute (10% in ethanol) phenol solution. Sham-operated rats had both kidneys exposed via the retroperitoneal incision and the renal nerves visualized but left intact. Renal sympathetic activity response to CSD In rats (SHR, n =6; Wistar, n =6) following implantation of the blood pressure catheter into the abdominal aorta and closure of the midline incision [33] , the right kidney was exposed via a retroperitoneal incision. Using a fine round-tipped glass hook, the renal nerve was freed from the surrounding connective tissue and a small patch of parafilm was slipped underneath to prevent fluid ingress. The nerve was passed over the electrodes from a sympathetic nerve activity telemeter (Model TR46SP, Telemetry Research Ltd., Auckland, New Zealand), carefully fixed in place using sutures, and then isolated from surrounding tissue with silicone elastomer (Kwik-Sil, WPI Inc.). A polyurethane catheter (0.033 in (~0.84 mm) outer diameter (OD); 0.014 in (~0.36 mm) inner diameter (ID); Micro-Renathane, Braintree Scientific) was implanted into the left femoral vein, connected to a transcutaneous port between the scapulae and flushed every 2–3 days with saline-containing heparin (100 U ml −1 ) and penicillin G (2,000 U ml −1 ) solution [11] . On days −2 and 8, the venous lines were connected and solutions of phenylephrine (0.1 mg ml −1 ) and sodium nitroprusside (0.1 mg ml −1 ) were infused i.v. to obtain ramp increases in arterial pressure of 1–2 mm Hg s −1 between ~60 and 180 mm Hg. These data were then used to generate 5-parameter sigmoidal regression baroreflex function curves. A brief sodium cyanide bolus (NaCN, 100 μl 0.04% i.v.) was given to stimulate peripheral chemoreceptors. The ‘zero’ level of renal sympathetic activity (RSA) was assessed after ganglionic blockade using hexamethonium tartrate (100 μl, 10 mg ml −1 i.v.). To assess any tonic activity generated by the CB, hyperoxia was used to ‘silence’ the CBs by briefly placing their cages into a plexiglass box connected to a 100% oxygen source on day −1. Arterial pressure was recorded 24 h per day, whereas RSA was recorded for 60 min at approximately the same time each day when animals were observed to be resting quietly. Arterial pressure and RSA signals were sampled at 500 Hz using an analogue-digital data acquisition card (PCI 6024E National Instruments, Austin, Texas) and continuously displayed by a data acquisition programme (Universal Acquisition 11, University of Auckland, Auckland, New Zealand). HR was derived from the arterial pressure waveform. The RSA signal was amplified, filtered between 50 and 5,000 Hz, full-wave rectified and integrated using a low-pass filter with a 20-ms time constant. At least 7 days were allowed for recovery before a 3-day baseline period was recorded. Arterial pressure and HR were recorded for 24 h a day. To avoid movement artefact, RSA was recorded for an hour at the same time each day, whereas the rats undisturbed in their home cage were observed to be quiescent. On days −2 and 7, rats were exposed to a brief burst of HF noise, which produces a stress increase in RSA. The magnitude of this response was used to check that the RSA signal remained viable and responsive throughout the experiment. Renal excretory function Rats were housed in metabolic cages with free access to water and food for 24 h. Blood was withdrawn from the tail vein. Plasma and urine creatinine were measured by improved Jaffe method with the commercially available QuantiCrom Creatinine Assay Kit (DICT-500, Universal Biologicals, Cambridge, UK) [58] . Creatinine clearance was estimated as (urinary creatinine ((μmol l −1 ) × volume urine produce in 24 h (ml))/(plasma creatinine (μmol l −1 ) × 1,440 (min)). Urinary albumin was measured by the improved bromocresol green (BCG) method [59] with the commercially available Albumin Assay (Randox Laboratories Ltd, Crumlin, UK) and the total protein was measured by the Lowry method [60] with the DC Protein Assay Kit (Bio-Rad Laboratories Ltd., Hemel Hempstead, UK). Urinary sodium was measured using an ion-selective electrode (Cole-Parmer, London,UK). Renal excretory function was assessed over a 24-h period before (day −2) and after (day 28) CSD ( n =6) or sham ( n =6) surgery. Renal noradrenaline content The left kidneys were crushed in liquid nitrogen and homogenized in an extraction buffer (0.01 M HCl, 1 mM EDTA, 4 mM sodium metabisulphite). Samples were centrifuged (8,000 r.p.m. for 30 min) and the supernatant protein concentration was determined by DC Protein Assay Kit (Bio-Rad Laboratories Ltd, No 500-0112). Tissue noradrenaline content was assessed by enzyme-linked immunosorbent assay (Alpco Diagonstics, USA) and normalized to protein concentration. FACS analysis of cellular inflammation Analysis of T cells in vascular homogenates of the aorta and brainstem was performed using fluorescence-activated cell sorting (FACS). To analyse leukocytes in the aorta and brain, tissue was digested using collagenase type IX (125 μ ml −1 ); collagenase type IS (450 U ml −1 ) and hyaluronidase IS (60 U ml −1 ) dissolved in 20 mM HEPES–PBS buffer for 30 min at 37 °C, during continuous agitation. The dissolved tissue was then passed through a 70-m sterile filter (Falcon, BD Biosciences), yielding a single-cell suspension. An additional step was applied for brain tissue using a 30/70% percoll gradient to separate out the mononuclear cell layer. All cells were then washed twice with FACS buffer (0.5% BSA in PBS) then counted, stained and analysed using multi-colour flow cytometry [61] . Antibodies (BD Biosciences) used for staining were as follows: V450 anti-CD45 and PE anti-CD3. After immunostaining, cells were resuspended in FACS buffer (0.5% BSA in PBS) and analysed immediately on a LSR-II flow cytometer with DIVA software (Becton Dickinson). Data were analysed with FlowJo software (Tree Star Inc., Ashland, Oregon, USA). In situ working heart–brainstem preparation As described originally [62] , animals were anaesthetized deeply (halothane), heparinized (1,000 units, intraperitoneal), bisected below the diaphragm and decerebrated pre-collicularly. Anaesthesia was terminated. Preparations were transferred to a recording chamber and a double lumen cannula was placed into the descending aorta for retrograde perfusion with a Ringer solution containing in mM NaCl (125), NaHCO 3 (24), KCl (3), CaCl 2 (2.5), MgSO 4 (1.25), KH 2 PO 4 (1.25), and D -glucose (10). Ficoll (molecular weight: 20,000; 1.25%) was added as an oncotic agent and the perfusion solution was saturated with 95% O 2 -5% CO 2 (pH, 7.35–7.4; osmolality 290±5 mosm±kg H2O −1 at 31 °C). Perfusion pressure was maintained between 60 and 80 mm Hg with additions of arginine vasopressin (200–400 pM, Sigma). A muscle relaxant, vecuronium bromide (4 μg ml −1 ; Organon Teknica, Cambridge, UK) was added to the perfusate. Recordings from the phrenic, lumbar sympathetic nerves and iCSN were made simultaneously using custom bipolar glass suction electrodes. Signals were amplified ( × 20k), filtered (60–3,000 Hz), rectified and integrated (50 ms time constant), and the noise level (obtained at the end of the experiment) was subtracted. Phrenic-triggered averaging of integrated sympathetic activity (over 10 phrenic cycles) allowed peak-to-trough amplitudes of the respiratory-related sympathetic burst to be measured. The Traube–Hering waves were also analysed using phrenic-triggered averaging. Cardiovascular responses to CSD and RD Radio-telemeters (PA-C40, Data Sciences Inc., St Paul, Minnesota, USA) were implanted as described before [33] , [34] . After 7 full days of recovery, 4 days of baseline arterial pressure was recorded before the first surgical intervention (All SH rats: CSD, n =7; sham–CSD n =7; RD, n =6; sham–RD n =6). Twenty-one days after CSD/sham–CSD, RD surgery was performed; conversely, 14 days after RD/sham–RD, CSD surgery was performed. Arterial pressure was recorded for 5 min every hour, 24 h per day using Hey Presto software, and HR and respiratory rate were derived from the arterial pressure waveform [33] . The data shown for cardiovascular parameters and ventilatory frequency represent daily averages from these 5-min periods. On the final day of the experiment, rats were euthanized (sodium pentobarbital 40 mg kg −1 , intraperitoneal) and the kidneys were extracted, weighed and frozen in liquid nitrogen for a noradrenaline assay. The aorta was removed for FACS and analysis of cellular inflammation (see below). Power spectral analysis Power spectral density was computed using purpose-written software [33] . The following frequencies were calculated in normalized units: <0.27 Hz (very low frequency), 0.27–0.75 Hz (LF) and 0.75–3.3 Hz (HF). The ratio of the LF to the HF component was used as an indicator of cardiac sympatho-parasympathetic balance. Spontaneous baroreflex gain was computed and respiratory rate was inferred from the peaks of respiratory modulation of the systolic pressure frequency spectrum. Data analysis From the arterial pressure waveform, values for systolic, diastolic, mean pulse pressure, HR and respiratory rate were derived. RSA is expressed as a percentage, where 100% is the average integrated value across the baseline period. Values are presented as mean±s.e.m. except where stated. Data were compared between baseline and CSD, and where applicable, RD time points, by repeated measures two-way analysis of variance, were followed where appropriate by the Holm–Sidek post hoc multiple comparison test. Differences within or between groups with P -values of <0.05 were considered significant. How to cite this article: McBryde, F. D. et al . The carotid body as a putative therapeutic target for the treatment of neurogenic hypertension. Nat. Commun. 4:2395 doi: 10.1038/ncomms3395 (2013).